Identification of high-quality cancer prognostic markers and metastasis network modules Early detection of various types of cancer before they spread would greatly aid clinicians. Prognostic biomarkers may help to improve the capacity to predict whether a patient's cancer is going to recur after surgical removal. Traditionally, clinical factors such as age and tumour grade have been used to assess prognosis; however, they have poor predictive power. As such, poor predictions of cancer recurrence lead to the overtreatment of many cancer patients. For example, 70–80% of lymph node-negative breast cancer patients may undergo adjuvant chemotherapy when it is, in fact, unnecessary [1] . In addition, almost 60–75% of women with early-stage breast cancer undergo a toxic therapy from which they will not receive any benefit, but instead will experience only side effects [2] . Therefore, it is essential to identify gene markers that are able to accurately identify low-risk cancer patients who do not require adjuvant chemotherapy. Genome-wide expression profiles that assess the risk of recurrence offer the possibility of more precisely defining clinical outcomes in cancer. Several predictors such as intrinsic-subtype classifiers [3] , the recurrence-score model [4] , the 70-gene signature [5] , the wound-response gene expression signature [6] and the ratio of the levels of expression of two genes [7] , which are largely based on an unsupervized analysis of breast tumour gene expression profiles ('one-step-clustering' approach), have been developed for breast cancer. However, these predictors have intermediate predictive power at best (accuracies below 70%) [8] , and they cannot be used across other patient cohorts. Recently developed stromal gene signature [9] and network-based gene signatures [10] , [11] showed some level of robustness. However, the accuracies of their predictions are still lower than 80%. Thus, researchers have struggled to identify robust and highly accurate prognostic biomarkers, not only for breast tumours but also for other types of cancers, during the past decade. The ITRANSBIG Consortium ( http://www.breastinternationalgroup.org ) suggests that, to be clinically practicable, low-risk patients should be associated with 10-year overall survival probabilities of at least 88% and 92% for ER+ and ER− tumours, respectively. Thus far, only Oncotype DX, a set of 21 cancer genes, has been shown clinically to be able to predict low-risk breast cancer patients with such a high degree of accuracy (>90%) [12] . However, Oncotype DX is only applicable to one clinical subtype of breast cancer patients (that is, Stage I/ER+ tumours). Moreover, the method by which the 21 genes of the Oncotype DX were generated cannot be applied to other breast cancer subtypes or other cancer types. Through an integrative analysis of a human signalling network and the output of the large-scale sequencing of tumour genomes, we previously showed that alterations of tumour suppressor genes (for example, p53 signalling) are essential in cancer development and progression [13] . Mutation of tumour suppressor genes often increases genome instability, which in turn induces genomic alterations such as rearrangements, chromosomal fragment amplifications and deletions [14] . Therefore, tumour cells often have many more 'passenger signals' than other types of cells, which means that the variability of gene expression profiles between individual tumours can be extremely high, and the 'real' cancer gene expression signals may be buried in these highly varied profiles. These insights suggest that the current marker identification method of the 'one-step-clustering' of microarray profiles of 'good' and 'bad' tumours captures numerous 'passenger signals' and renders markers derived from this approach less robust and accurate. On the basis of these insights, we developed a new algorithm: Multiple Survival Screening (MSS). By applying MSS to breast tumours, we discovered six and three marker sets for ER+ and ER− subtypes, respectively. We identified low-risk cancer patients with high rates of accuracy (that is, 87–96% and 88–100% in eight patient cohorts containing 1,375 samples for good outcomes in the low-risk groups of ER+ and ER− subtypes, respectively). Moreover, MSS is applicable to other cancer types and subtypes for the identification of prognostic or drug response biomarkers. Finally, an integrative network analysis of these gene signatures and breast cancer driver-mutating genes in a protein interaction network allowed the identification of several metastasis network modules in which each module contains the genes of one signature and their directly interacting partners that are cancer driver-mutating genes. We show that these network modules are repeatedly used in most breast tumours by the molecular mechanisms of cancer metastasis. Most of the multiple prognostic makers are not robust We have demonstrated that those genes the expressions of which are correlated with patient survival have a better chance of being associated with metastasis (see Supplementary Fig. S1 and Supplementary Methods ). However, tumour heterogeneity prevents the identification of robust cancer biomarkers. It is unknown to what extent tumour heterogeneity affects the robustness of gene signatures. To answer this question, we carried out a simulation study. We performed a genome-wide screening of genes, the expressions of which are correlated with patient survival, by conducting survival analysis (referred to as survival screening here) as described previously [13] , for the data sets from the cohorts of Wang et al . [15] , Chang et al . [6] and van 't Veer et al . [5] (see Methods ). As a result, we obtained three gene lists containing 1,755, 3,233 and 1,834 genes, respectively. We found 113 genes that are common among the three gene lists. 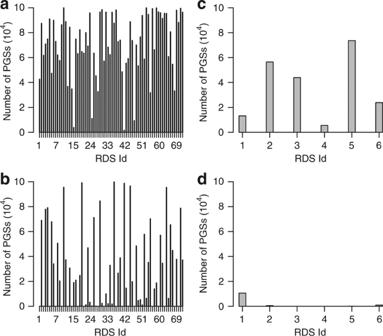Figure 1: The number of passed gene sets (PGSs) in the random data sets. The random microarray data sets (RDSs) generated from (a) the Chang data set and (b) the Wang data set. The number of PGSs in the six ER+ random data sets (c) and the six ER− random data sets (d) generated from the Wang data set. A PGS is a gene set with a survival screeningP-value of <0.01 when the gene set is used to perform survival screen analysis on an RDS. A total of 49 of the 113 genes are related to cancer hallmarks (that is, genes belonging to cancer-related Gene Ontology (GO) terms, Table 1 ). How transferable is a signature derived from one data set when applied to another? To answer this question, we generated 72 virtual data sets, called random microarray data sets (RDSs), by randomly selecting 74 samples from the Chang data set. Each RDS was required to maintain the same ratio of 'good' and 'bad' tumours as that of the original set, with <30% sample overlap among the RDSs. Next, we generated 10 5 distinct random gene sets (RGSs) by randomly selecting 30 genes from the 49 genes mentioned above. We performed a survival screen using each RGS against each RDS. For each RDS, we counted the number of gene sets (each referred to as a 'passed gene set', PGS) the survival screening P -value of which is <0.01. Table 1 Selected gene groups used to generate the 1 million random gene sets. Full size table Despite the fact that RDSs were subsets of the same original cohort, the number of PGSs varied greatly from one RDS to another ( Fig. 1a ). We extended the same analysis to the Wang data set and even greater variability was observed ( Fig. 1b ). As shown in Figure 1 , some RDSs can have tens of thousands of PGSs, that is, gene sets that seem to be predictive for a particular virtual cohort. However, the large variability in the number of PGSs shows that one can have tens of thousands of PGSs for one RDS that are not transferable to another RDS. We conclude that most of the PGSs are not robust (that is, the predictive power of one PGS for one RDS can be easily lost in another RDS). It should be noted that all of these RDSs are subsets of their original data sets, which means that, in this simulation study, we excluded the potential effects of variability of the usage of different microarray platforms and experiments performed by different laboratories (that is, different laboratories may have varied the procedures of sample handling, preparation of mRNA and hybridization). These results illustrate why the commonly used approach of using 'one-step-clustering' is unable to generate robust gene signatures. Different combinations of tumour samples in one data set and the extremely large individual variability of tumour gene expression profiles result in 'passenger signals' that can effectively drown out the 'real' gene signatures in the noise. Figure 1: The number of passed gene sets (PGSs) in the random data sets. The random microarray data sets (RDSs) generated from ( a ) the Chang data set and ( b ) the Wang data set. The number of PGSs in the six ER+ random data sets ( c ) and the six ER− random data sets ( d ) generated from the Wang data set. A PGS is a gene set with a survival screening P -value of <0.01 when the gene set is used to perform survival screen analysis on an RDS. Full size image Cancer subtypes can provide a way to improve robustness by providing a means of first classifying samples for which specific signatures can be obtained. For example, breast cancer is clinically divided into ER+ and ER− subtypes [17] . The mixture of different subtypes in a single breast cancer data set could confound attempts to identify gene signatures suitable for the entire set. To exemplify this, we generated six RDSs that contain only ER+ samples and another six RDSs that contain only ER− samples using the Wang data set. We performed survival screens on these RDSs using the 10 5 RGSs mentioned above. Surprisingly, no PGSs were found in five of the six ER− RDSs, whereas more than 5,000 PGSs were found in all ER+ RDSs ( Fig. 1c,d ). These results suggest that we should identify specific gene signatures for ER+ and ER− tumours separately. Other types of cancer might have no known subtypes. For these cases, we developed a method to find clinical/molecular features that are potentially useful for identifying subtypes as a first step for classifying samples (see Supplementary Methods ). On the basis of these insights, we developed a new algorithm, MSS, for identifying robust and highly accurate biomarkers from gene expression profiles of tumours (see Supplementary Software ). 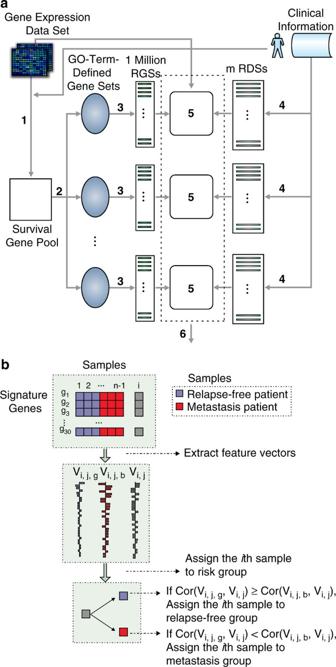Figure 2: Scheme of the algorithms. (a) Multiple Survival Screening (MSS). Numbers in bold refer to the main steps in the MSS algorithm.mandnrepresent numeric numbers. (1) Generate a survival gene list by a genome-wide survival analysis of the training set (T1 set). (2) Assign survival genes to non-exclusive GO (Gene Ontology)-term-defined gene sets on the basis of cancer-related GO terms. (3) Generate 1 million random gene sets (RGSs) with 30 genes taken from the GO-term-defined set. (4) Generate 36 random data sets (RDSs) from the T1 set (maintaining the same ratio of 'good' and 'bad' tumours as in the original T1 set). (5) For each RGS–RDS pair, calculate the survival screeningP-value of the RGS. (6) Identify the RGSs that are predictive (P-value <0.05). The top 30 most frequent genes among the predictive RGSs are used as a potential gene signature. (b) Testing the National Research Council (NRC-j,j=1, 2, 9) gene signatures. A feature vector, Vi,j, based on the expression levels of signature genes in NRC-j is calculated for each samplei. Leave-one-out testing is then used to determine the ability of the gene signature to classify each sample. For each sampleileft out, the nearest-shrunken-centroid method is used to calculate 'average' feature vectors, Vi,j,gand Vi,j,b, for the 'good' or 'bad' tumour samples, respectively, in the remainingn−1 samples. Pearson's correlation coefficients Cor (Vi,j,g, Vi,j) and Cor (Vi,j,b, Vi,j) are then used to assign sampleito that group in which the 'average' feature vector is more correlated to that of samplei. Details of the algorithms can be found inSupplementary Methods. Figure 2a shows a scheme of the method (see Supplementary Methods ). The algorithm was developed for searching biomarker genes with optimized combinatorial effects (that is, in cases in which the effect is not purely additive but combinatory and nonlinear). As a proof of concept, we applied the algorithm to breast cancer patients. Figure 2: Scheme of the algorithms. ( a ) Multiple Survival Screening (MSS). Numbers in bold refer to the main steps in the MSS algorithm. m and n represent numeric numbers. (1) Generate a survival gene list by a genome-wide survival analysis of the training set (T1 set). (2) Assign survival genes to non-exclusive GO (Gene Ontology)-term-defined gene sets on the basis of cancer-related GO terms. (3) Generate 1 million random gene sets (RGSs) with 30 genes taken from the GO-term-defined set. (4) Generate 36 random data sets (RDSs) from the T1 set (maintaining the same ratio of 'good' and 'bad' tumours as in the original T1 set). (5) For each RGS–RDS pair, calculate the survival screening P -value of the RGS. (6) Identify the RGSs that are predictive ( P -value <0.05). The top 30 most frequent genes among the predictive RGSs are used as a potential gene signature. ( b ) Testing the National Research Council (NRC-j, j =1, 2, 9) gene signatures. A feature vector, V i,j , based on the expression levels of signature genes in NRC-j is calculated for each sample i . Leave-one-out testing is then used to determine the ability of the gene signature to classify each sample. For each sample i left out, the nearest-shrunken-centroid method is used to calculate 'average' feature vectors, V i,j,g and V i,j,b , for the 'good' or 'bad' tumour samples, respectively, in the remaining n −1 samples. Pearson's correlation coefficients Cor (V i,j,g , V i,j ) and Cor (V i,j,b , V i,j ) are then used to assign sample i to that group in which the 'average' feature vector is more correlated to that of sample i . Details of the algorithms can be found in Supplementary Methods . Full size image Gene signatures for the ER+ subtype To apply the algorithm to breast cancer ER+ patients, we extracted microarray data for all the ER+ samples (209 samples, referred to as the training set (T1 set)) from the Wang data set. Genome-wide gene survival screening for the T1 set yielded 1,522 genes the P -values of which were <0.05. We then performed GO annotation of the 1,522 genes using cancer-related GO terms. We generated 36 RDSs from the T1 set. For each selected gene group, we applied the MSS algorithm to the 36 RDSs. ( Supplementary Tables S1 and S2 list the GO terms and parameters used in the analysis.) To assess the reproducibility and stability of gene signatures for each selected gene group, we generated another 1 million distinct RGSs (that is, no RGS in the second set seems in the previous 1 million RGSs) and re-ran the survival screening and gene ranking processes of the algorithm. Of the top 30 genes, 29 were common between the two independent runs for the cell cycle gene group. A similar reproducibility between independent runs was obtained for the apoptosis (28 of 30) and immune response (28 of 30) gene groups. However, the results from the other selected gene groups were not as reproducible. We therefore obtained the first batch of marker sets from the cell cycle, apoptosis and immune response gene groups, defined as National Research Council (NRC) gene signatures NRC-1, -2 and -3 (see Supplementary Data 1 ), respectively. We applied the nearest shrunken centroid classification [18] and the leave-one-out method ( Fig. 2b , see Supplementary Methods ) to evaluate the prognostic value of each ER+ gene signature (NRC-1, -2 and -3) in the T1 set and in eight other independent breast cancer cohorts ( Supplementary Table S2 ). The three signatures are able to distinguish 'good' and 'bad' ER+ tumours in both the training and testing sets ( Supplementary Fig. S2 ). In contrast, when we tested the top 30 genes from the non-reproducible gene lists, these lists often failed in the testing sets. These results highlight the robustness of the gene signatures generated by the MSS algorithm. To determine whether the combined use of the three gene signatures would result in a better prediction of patient outcome than the use of any one alone, we conducted combinatorial tests of the T1 set in two ways: (1) we appended the genes from the three NRC gene signatures to generate one meta-gene signature. The meta-gene signature was predictive, but no better than that of the three independent gene signatures ( Supplementary Table S3 ); and (2) we used each gene signature independently and assigned 0 or 1 (representing predicted good and poor outcomes, respectively) to the samples. By combining the predicted results of the three gene signatures, we were able to stratify the samples into three groups: low risk (assigned 0 by all three signatures), high risk (assigned 1 by all three signatures) and intermediate risk (the assignments of the three signatures were not in agreement). Interestingly, 89 and 91% of the low-risk and high-risk samples, respectively, were predicted correctly, but only 58% of the intermediate-risk samples were predicted so. We decided to identify more gene signatures that could be used to predict recurrence for the intermediate- and high-risk groups mentioned above. Towards this end, we re-ran the algorithm using the samples from intermediate- and high-risk groups of the T1 set, respectively. For the intermediate-risk group samples, we could not find additional gene signatures that were significantly better to stratify the samples. For the high-risk group samples, however, we obtained another three gene signatures, defined as NRC-4, NRC-5 and NRC-6. The parameters used for identifying these signatures are listed in Supplementary Table S1 . We next developed a diagnostic procedure for the ER+ samples using these six signatures ( Fig. 2b , see Supplementary Methods ). We validated the six signatures and the procedure in 1,182 ER+ samples from the eight independent breast cancer patient cohorts. As shown in Table 2 and Fig. 3 , combined use of the six signatures was able to stratify ER+ patients into low-, intermediate- and high-risk groups in both the training and testing sets. In particular, the accuracy of the low-risk group reaches 87–96% in these cohorts. Table 2 The accuracy of ER+ samples by combinatorial use of the NRC signatures. 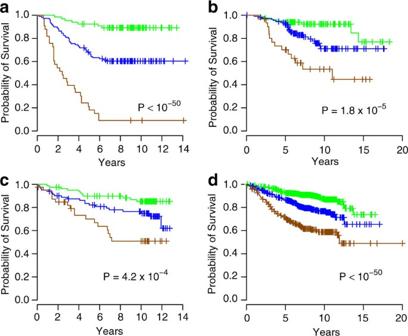Figure 3: Kaplan–Meier curves of the risk groups for ER+ patients with 10-year disease-free survival predicted by the combinatorial use of NRC-1 to NRC-6. (a) Wang cohort. (b) Chang cohort. (c) Miller cohort. (d) Metadata containing 1,009 ER+ samples from Affymetrix data sets minus the training set (Wang cohort). Green, blue and dark orange curves represent low-, intermediate- and high-risk groups, respectively.P-values were obtained from theχ2-test. Full size table Figure 3: Kaplan–Meier curves of the risk groups for ER+ patients with 10-year disease-free survival predicted by the combinatorial use of NRC-1 to NRC-6. ( a ) Wang cohort. ( b ) Chang cohort. ( c ) Miller cohort. ( d ) Metadata containing 1,009 ER+ samples from Affymetrix data sets minus the training set (Wang cohort). Green, blue and dark orange curves represent low-, intermediate- and high-risk groups, respectively. P -values were obtained from the χ 2 -test. Full size image Gene signatures for ER− samples To identify gene signatures for ER− samples, we ran the same algorithms using the 77 ER− samples from the Wang data set and obtained three gene signatures, NRC-7, NRC-8 and NRC-9. The parameters used for identifying these signatures are listed in Supplementary Table S1 . There are 25, 27 and 26 genes in common, respectively, between the two independent runs for each gene group that was used for generating NRC-7, NRC-8 and NRC-9. Theses results suggest that the signatures have high reproducibility. By combined use of the three signatures, we were able to stratify the ER− samples into low-, intermediate- and high-risk groups. Because the number of ER− samples is usually small, we combined the intermediate- and high-risk groups to form the high-risk group. We tested the predictive performance of NRC-7, -8 and -9 in the T1 set and in the five testing cohorts. Similar to ER+ signatures, ER− signatures also performed well, that is, 88–100% accuracy for low-risk groups in the testing sets containing 193 samples ( Table 3 , Fig. 4 and Supplementary Fig. S3 ). Table 3 The accuracy of ER− samples by combinatorial use of the NRC signatures. 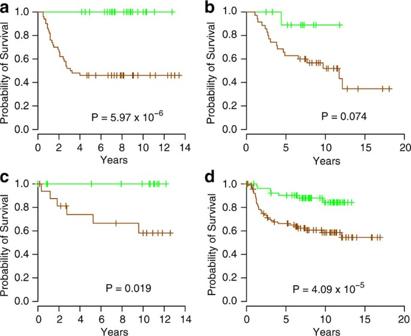Figure 4: Kaplan–Meier curves of the risk groups for ER− patients with a 10-year disease-free survival predicted by the combinatorial use of NRC-7 to NRC-9. (a) Wang cohort. (b) Chang cohort. (c) Miller cohort. (d) Metadata containing 146 ER− samples from Affymetrix data sets minus the training set (Wang cohort). Green and dark orange curves represent low- and high-risk groups, respectively.P-values were obtained using theχ2-test. Full size table Figure 4: Kaplan–Meier curves of the risk groups for ER− patients with a 10-year disease-free survival predicted by the combinatorial use of NRC-7 to NRC-9. ( a ) Wang cohort. ( b ) Chang cohort. ( c ) Miller cohort. ( d ) Metadata containing 146 ER− samples from Affymetrix data sets minus the training set (Wang cohort). Green and dark orange curves represent low- and high-risk groups, respectively. P -values were obtained using the χ 2 -test. Full size image NRC signatures derived metastasis network modules To understand why these NRC signatures perform well, we examined the relationships between signatures and breast cancer driver-mutating genes, which were obtained from literature curation and the large-scale sequencing of tumour samples, on a human protein interaction network (see Methods ). We mapped the NRC-1 signature genes, which represent cell cycle processes, and the breast cancer driver-mutating genes onto the human protein interaction network, and identified 33 breast cancer-mutating genes (referred to as NRC-1_driver_genes, Fig. 5 , see Supplementary Data 2 ), which are the direct interacting neighbours of NRC-1 signature genes. 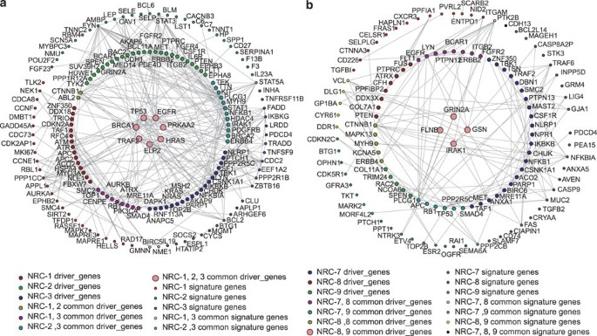Figure 5: Relationships between NRC signature genes and their driver-mutating genes in the protein interaction network. (a) For NRC-1, -2 and -3. (b) For NRC-7, -8 and -9. The largest spheres represent the common driver_genes from all the driver_gene sets, whereas the middle and small sizes of spheres represent driver_genes and signature genes, respectively. A driver_gene is a gene that is known as a breast cancer driver_mutating gene and the coding protein of which directly interacts with the protein coded by a signature gene. A common driver_gene or a common signature gene is a gene that is found in at least two driver_gene lists (that is, NRC-1 driver_genes and NRC-2 driver_genes) or in at least two signature gene lists (that is, NRC-1 and NRC-2), respectively. Figure 5: Relationships between NRC signature genes and their driver-mutating genes in the protein interaction network. ( a ) For NRC-1, -2 and -3. ( b ) For NRC-7, -8 and -9. The largest spheres represent the common driver_genes from all the driver_gene sets, whereas the middle and small sizes of spheres represent driver_genes and signature genes, respectively. A driver_gene is a gene that is known as a breast cancer driver_mutating gene and the coding protein of which directly interacts with the protein coded by a signature gene. A common driver_gene or a common signature gene is a gene that is found in at least two driver_gene lists (that is, NRC-1 driver_genes and NRC-2 driver_genes) or in at least two signature gene lists (that is, NRC-1 and NRC-2), respectively. Full size image Because NRC-1 is a cell cycle prognostic signature across patient cohorts, we hypothesized that NRC-1_driver_genes may be associated with the cell cycle process involved in cancer metastasis across patient cohorts. To test this hypothesis, we collected all proteins (referred as NRC-1_driver_neighbor genes) that are the direct interacting neighbours of not only NRC-1_driver_genes (33 genes) but also of cell cycle genes (using GO annotation) in which NRC-1 signature genes have been removed. We then performed survival analysis of NRC-1_driver_neighbour genes in the Wang, Chang and Miller cohorts. Interestingly, NRC-1_driver_neighbour genes significantly distinguished 'good' and 'bad' ER+ tumours in all the cohorts. These results suggest that in the context of cell cycle processes, the 33 NRC-1_driver_genes may be associated with metastasis across patient cohorts, and, furthermore, may be commonly used for metastasis in many ER+ samples. We further performed the above analyses 5,000 times but randomly picked 33 breast cancer-mutating genes each time (see Methods ) and showed that the 33 NRC-1_driver_genes are uniquely associated with metastasis in the context of cell cycle process ( P <0.018), suggesting that they are recurrently used for metastasis by many ER+ samples. Similar results were obtained by extending the above analysis to the gene signatures of NRC-2, -3 and -7- to -9 signatures ( Fig. 5 , see Supplementary Data 2 ). This indicates that each gene signature forms a network module with a unique driver-mutating gene set, which is used by the molecular programme of metastasis across many tumour samples. In this study, we developed the MSS algorithm using a semi-supervized approach and identified several breast cancer prognostic marker sets. These marker sets were validated and shown to be highly predictive in eight independent breast tumour microarray data sets. Compared with the existing signatures, NRC signatures reached both high predictive accuracies (87–96%, 88–100% for ER+ and ER− patients, respectively) and high robustness (tested in eight independent breast cancer cohorts containing 1,182 ER+ and 193 ER− samples). Network analyses of these signatures and of breast cancer driver-mutating genes identified several network modules involved in metastasis. Using a stimulation study, we showed that the predictive power of most of the gene signatures in one data set can be easily lost in another data set, suggesting that interpatient and intratumour heterogeneity has an important role in affecting the robustness of gene signatures. These insights indicate that the dominantly used concept/approach of 'one-step-clustering' of gene expression profiles is unable to generate robust gene signatures. This motivated the development of the MSS algorithm. The heart of MSS is the screening of randomized data sets using randomly generated gene combinations. The interactions of gene expression values within one predictive gene set are known to be nonlinear. Thus, the algorithm is preferable to simple clustering methods for identifying predictive gene signatures. Furthermore, the reproducibility and stability of gene signatures were evaluated and confirmed by performing another round of screening of multiple data sets and gene ranking. The results are encouraging and can be interpreted to mean that a core set of genes within a predictive gene signature preferentially interact with each other and are commonly used in the metastatic programme by many individual tumours. Data overfitting is always a challenge in biomarker discovery. There is a large input dimensionality (thousands of genes) and a paucity of patient samples (a few hundred is typical); thus, it is statistically plausible to have small subsets that are randomly correlated with any given desired outcome, irrespective of any biological functionality of the gene expression itself. As we mentioned earlier, there are many more 'passenger signals' in gene expression profiles than expected. Thus, the 'cancer driver-associated signals' are deeply buried in passenger signals. To cope with this problem, we targeted select genes in a biased manner, that is, by selecting those cancer-associated (cancer hallmark) genes the expression values of which are correlated with patient survival. By doing so, we minimized sparse correlations and the problem of overfitting. Genes in one cancer hallmark GO term may be expressed in a coordinated manner so that a subset of these genes could maintain the interactions of their expressions. Therefore, gene signatures derived from these GO terms most likely reflect cancer processes and are therefore more robust. Finally, to improve accuracy, we used the results of three predictive gene signatures combinatorially and showed that this strategy is able to significantly increase the predictive accuracy, especially in low-risk groups. Tumour progression and metastasis are distinct processes. Oncogenic transformation leading to tumour progression is not sufficient for metastatic competence. It is believed that many genetic and epigenetic events contribute to the metastatic path. Tumour genome sequencing provides a powerful approach for cataloguing cancer driver-mutating genes; however, it cannot distinguish those genes that are the drivers of tumour progression, metastasis or both. In this study, we have dissected several sets of driver-mutating genes for metastasis by integrative analysis of the human protein interaction network and prognostic signatures. NRC driver-gene sets show that most of these mutated genes are significantly enriched for signalling proteins ( P -values range from 3.5×10 −5 to 4.9×10 −11 ), whereas more than 40% of genes in the NRC signatures encode secreted and cell surface proteins ( Supplementary Data 1 ). These results suggest that each network module contains two parts: a set of NRC signature genes (that is, the 'modulated part'; these genes are dynamically modulated between 'good' and 'bad' tumours) and a unique set of cancer driver-mutating genes (that is, the 'mutating part'; one or more genes are mutated and hijack normal cell signalling events) that are the direct protein interacting partners of the signature genes. Taken together, we believe that, during metastasis, one or more genes of the 'mutating part' get mutated and alter normal cell signalling, whereas the genes of the 'modulated part' are dynamically modulated between 'good' and 'bad' tumours. Thereafter, the genes from the 'mutating part' are rewired (that is, the interaction between the proteins from the two parts is changed because of the high or low expression of genes). More importantly, the enrichment of secreted and cell surface proteins in the 'mutating part' suggests an intensive communication between network modules and tumour microenvironments. This conclusion supports the notion that the nature of the metastatic process is such that cancer cells need to communicate with the tumour microenvironment and overcome hurdles for cell motility, circulation and the infiltration of distant organs. The mediators of metastasis (that is, the 'mutating part' of the network modules) may also have dual functions that provide both a local advantage for malignant progression in the primary tumour and a distal advantage for metastasis. Recently, p53 was shown to have both functions [19] . For the ER+ and ER− subtypes, we have identified three metastasis network modules representing three different cell signalling processes, suggesting that a higher order of coordination exists between these cellular processes. Indeed, many interacting links can be found among the genes of the three processes/network modules (that is, cell cycle, apoptosis and immunological responses for the ER+ subtype, and apoptosis, cell proliferation and cell adhesion for the ER− subtype). Furthermore, the fact that NRC signatures have predictive power across patient cohorts suggests that these network modules are collaborated and repeatedly used in many breast tumour samples by the molecular programme of metastasis. In addition, the metastasis driver gene sets of apoptosis often contain many genes in common with those representing other key metastasis signalling processes. This observation is in agreement with the finding that, during evolution, apoptotic proteins tend to integrate into other signalling pathways [20] . By examining the GO terms of NRC signatures for the ER+ and ER− subtypes, we found that only one GO term or gene group (apoptosis) is common between the two subtypes (NRC-3 for ER+ and NRC-7 for ER−). However, the gene sets of the two apoptotic groups have only a single gene in common, and the network modules are also different between the two subtypes. These results suggest that different molecular metastatic programmes are used in the ER+ and ER− subtypes, respectively. In summary, we showed that the concept of 'one-step-clustering' of gene expression profiles, which has been dominantly used in the past decade, is not suitable for generating robust gene signatures. Therefore, we developed an algorithm for identifying prognostic markers that can be used in combination to stratify breast cancer patients into groups with different risk ranks. The NRC signature sets showed high predictive accuracy, especially for low-risk patient groups. More importantly, the algorithm can be applied to other cancer types and subtypes. Our approach might provide a framework for discovering robust and reproducible gene signatures for specific phenotypes, such as clinical outcome, drug response or other disease features. Finally, a network analysis of NRC gene signatures and breast cancer driver-mutating genes identified several network modules that are recurrently used in breast tumours by the molecular programme of metastasis. Each network module contains a core set of driver-mutating genes, the mutation of which alters cell signalling, and another set of genes of one NRC signature the expressions of which change dynamically, rewiring the mutating genes (for cell signalling) and being extensively involved in cell communications between tumours and their microenvironments. Breast cancer data sets The breast cancer microarray data sets used were from Wang et al . [15] (Wang cohort or data set, Affymetrix arrays), Chang et al . [6] (Chang cohort or data set, cDNA arrays), van 't Veer et al . [5] (van 't Veer cohort or data set, cDNA arrays), Miller et al . [21] (Miller cohort or data set, Affymetrix arrays) and from several other Affymetrix array data sets with the following NCBI GEO ( http://www.ncbi.nlm.nih.gov/geo/ ) IDs: GSE11121 , GSE1456 , GSE6532 , GSE9151 , GSE7378 and GSE12093 . Supplementary Table S2 summarizes the number of ER+ and ER− samples for each data set. The Wang data set and the van 't Veer cohort were used as the T1 set (we tested whether adding an extra data set, the van 't Veer cohort, to RDSs generated from the Wang cohort could improve the performance of MSS; we did not observe significant improvements), whereas other cohorts were used as the testing sets. The Chang cohort contains samples from the van 't Veer cohort. When testing the Chang cohort, we removed the samples in common with the van 't Veer cohort. Samples without clinical information were dropped and the gene expression data were z -score normalized. Human protein interaction network The data for constructing the human protein interaction network were downloaded from the I2D database [22] . Breast cancer driver-mutating genes Breast cancer driver-mutating genes were obtained from COSMIC (Catalogue Of Somatic Mutations In Cancer, http://www.sanger.ac.uk/genetics/CGP/cosmic/ ) and Sjoblom et al . [23] Microarray metadata normalization Except for the Chang and van 't Veer data sets, the data sets used are Affymetrix arrays. We combined a metadata set for all ER+ samples from the testing sets generated using Affymetrix platforms. To do so, Affymetrix expression data were analysed using the MAS5.0 algorithm. Subsequently, data were log2 transformed, the values of the probes belonging to the same gene were averaged and then median-centred across arrays. Finally, gene expression data were z -score normalized across arrays. A similar procedure was applied to generate a metadata set for ER− samples. Survival analysis of NRC_driver_neighbour genes We use NRC-1_driver_genes to illustrate this analysis. NRC-1_driver_genes are the breast cancer driver-mutating genes that are also direct interacting partners of NRC-1 signature genes. We identified 33 NRC-1_driver_genes. To perform survival analysis, we collected all proteins (referred to as NRC-1_driver_neighbour genes) from the protein interaction network that are direct interacting neighbours of the NRC-1_driver_genes and also members of the cell cycle gene set from which the NRC-1 signature genes were removed. We tested the predictive power of NRC-1_driver_neighbour genes in the Wang, Chang and Miller data sets. To do so, we first performed t -tests of the expression values of each NRC-1_driver_neighbour gene between the 'good' and 'bad' tumours of the ER+ samples of the three cohorts. To increase the number of cell cycle genes of the NRC-1_driver_neighbour genes for the survival analysis, we selected those genes the P -values of which are <0.5 and 0.2 (we used these two cutoffs and found that the trends were the same regardless of the cutoffs) to perform the survival analysis for the ER+ samples of each cohort. We then obtained P -values for the NRC-1_driver_neighbour genes P c-1-NRC1 , P c-2-NRC1 and P c-3-NRC1 for each cohort. The same method was applied to NRC-2, -3, -7, -8 and -9 gene signatures. For NRC-7, -8 and -9, the ER− samples of the three cohorts were used. Randomization tests for the driver_neighbour genes We use the 33 NRC-1_driver_genes to illustrate the test. To perform the randomization tests, we randomly selected 33 breast cancer driver-mutating genes that were mapped onto the protein interaction network. Using the survival analysis method mentioned above, we selected the 33-driver_neighbour genes and performed the survival analysis in the ER+ samples of the three cohorts (the training and two testing sets: Chang and Miller data sets) and obtained P -values, P c-1-random , P c-2-random and P c-3-random , for each cohort , respectively. We tested the null hypothesis, P c-1-random >= P c-1-NRC1 , P c-2-random >= P c-2-NRC1 and P c-3-random >= P c-3-NRC1 , by performing 5,000 randomization tests and calculating the P -value. How to cite this article: Li, J. et al . Identification of high-quality cancer prognostic markers and metastasis network modules. Nat. Commun. 1:34 doi: 10.1038/1033 (2010).